Bacterial killing via a type IV secretion system Type IV secretion systems (T4SSs) are multiprotein complexes that transport effector proteins and protein–DNA complexes through bacterial membranes to the extracellular milieu or directly into the cytoplasm of other cells. Many bacteria of the family Xanthomonadaceae, which occupy diverse environmental niches, carry a T4SS with unknown function but with several characteristics that distinguishes it from other T4SSs. Here we show that the Xanthomonas citri T4SS provides these cells the capacity to kill other Gram-negative bacterial species in a contact-dependent manner. The secretion of one type IV bacterial effector protein is shown to require a conserved C-terminal domain and its bacteriolytic activity is neutralized by a cognate immunity protein whose 3D structure is similar to peptidoglycan hydrolase inhibitors. This is the first demonstration of the involvement of a T4SS in bacterial killing and points to this special class of T4SS as a mediator of both antagonistic and cooperative interbacterial interactions. Bacterial cells are continuously interacting with other bacterial and eukaryotic cells in a relentless battle for survival. These interactions have driven the evolution of several mechanisms by which they quickly deploy proteinaceous and nucleic acid effectors that manipulate the behaviour of the target organism, often resulting in growth inhibition or death [1] , [2] , [3] , [4] , [5] , [6] . Distinct among these mechanisms are the type III, type IV and type VI secretion systems (T3SS, T4SS and T6SS, respectively) that are all capable of transferring proteins, and in the case of the T4SS, protein–DNA complexes, directly into neighbouring cells in a contact-dependent manner [1] , [2] , [3] . All three of these systems have been shown to be able to inject virulence factors into eukaryotic hosts, but only the T6SSs have been shown to deliver lethal toxins into bacterial cells [7] . T4SSs are perhaps the most versatile of the macromolecular transport systems, being essential for host colonization by many medically important microbes [8] , [9] , [10] , [11] , [12] , [13] , the horizontal transfer of genetic material between bacteria and from bacteria to plants [2] as well as the special cases of the Helicobacter pylori DNA uptake [14] and Neisseria gonorrhoeae DNA release [15] systems. The prototypical T4SS is that of the plant pathogen Agrobacterium tumefaciens that uses its Vir system to cause tumours in most dicotyledonous species [16] . T4SSs are generally made up of a core set of 12 proteins, named VirB1–VirB11 plus VirD4 with a structural organization that is only now being elucidated: (i) a set of three cytoplasmic ATPases (VirB4, VirB11 and VirD4) that energize secretion; (ii) a periplasmic core complex made up of 14 repeats of a VirB7–VirB9–VirB10 trimer, in which VirB10 inserts into both inner and outer membranes and VirB7 is an outer membrane lipoprotein; (iii) an inner membrane complex that includes VirB3, VirB6 and VirB8; (iv) an extracellular pilus formed by VirB2 and VirB5; and (v) the periplasmic transglycosylase VirB1 (refs 2 , 17 , 18 , 19 ). Many bacteria of the family Xanthomonadaceae, which occupy diverse environmental niches, carry a T4SS with unknown function but with several characteristics that distinguishes it from other T4SSs [20] , [21] . One of these distinguishing features is that the Xanthomonas citri (Xac) VirD4 protein (VirD4 XAC2623 ), a homologue of the coupling protein that recruits effectors to the T4SS for secretion [2] , interacts with a set of uncharacterized Xanthomonas VirD4-interacting proteins (XVIPs) that all contain a conserved C-terminal domain termed XVIPCD (XVIP-conserved domain) [20] . In this study, we show that these XVIPs are toxins secreted by the Xanthomonas T4SS, that secretion is dependent on the XVIPCD and that this special T4SS is used by Xanthomonas to kill other bacterial cells, thereby providing a competitive growth advantage in mixed bacterial communities. A hypothesis for a new physiological role for a T4SS The Xac XVIPs are highly diverse in size and architecture and lack a canonical signal sequence. Six Xac XVIPs (XAC0466, XAC0574, XAC1918, XAC2609, XAC2885 and XAC3634) are predicted to act within the periplasm as peptidoglycan (PG)-binding proteins, PG glycohydrolases, lytic transglycosylases, PG peptidases or lipases ( Fig. 1a ). Furthermore, the genes of these proteins, plus one other containing an HExxH metallopeptidase motif (XAC0096), are found downstream to, and potentially co-transcribed with, genes that code for proteins with unknown functions with predicted lipoprotein signal peptides that are expected to localize them within the bacterial periplasm ( Fig. 1 ). One XVIP (XAC2609) has a complete PG-binding domain (residues 219–280) and a region (residues 30–120) with similarity to the catalytic region of proteins of glycoside hydrolase family 19 (GH19) that possess chitinase- or lysozyme-like activities [22] ( Fig. 1 ). XAC2609 has been shown to interact with the putative periplasmic lipoprotein XAC2610 and both are coded by genes within the Xac chromosomal T4SS vir locus [20] . These characteristics are very similar to those observed for certain T6SS effectors with hydrolytic activities against conserved PG and phospholipid components of the bacterial cell wall and their cognate immunity proteins [23] , [24] . On the basis of these observations, one hypothesis is that the Xac T4SS could secrete toxins participating in toxin–immunity protein systems. 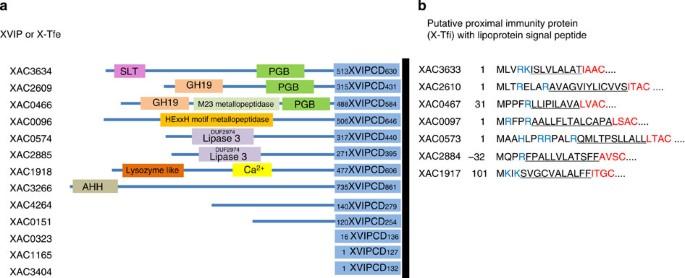Figure 1: Xac X-Tfe proteins and their respective putative X-Tfi immunity proteins. (a) Gene names and domain architectures of the 13 Xac X-Tfes. All these proteins contain aXanthomonasVirD4-interacting protein conserved domain (XVIPCD)20. PGB, peptidoglycan-binding domain; GH19, glycohydrolase family 19; SLT, soluble lytic transglycosylase; Ca2+, Ca2+-binding domain; AHH, putative nuclease domain. (b) Gene names of putative lipoprotein signal peptide-containing Xac immunity proteins (X-Tfis) and sequences of the putative lipoprotein signal peptides. All seven of these genes are upstream of, and potentially co-transcribed with, the neighbouring X-Tfe gene. Lipoprotein signal peptides are characterized by an N-terminal basic region (basic residues coloured blue), a central hydrophobic region (underlined) followed by an [LVI]-[ASTVI]-[AGS]-C lipobox motif (red)68. Also indicated are the positions of the putative translation initiation codons relative to those found in the original annotation of the Xac genome69. Figure 1: Xac X-Tfe proteins and their respective putative X-Tfi immunity proteins. ( a ) Gene names and domain architectures of the 13 Xac X-Tfes. All these proteins contain a Xanthomonas VirD4-interacting protein conserved domain (XVIPCD) [20] . PGB, peptidoglycan-binding domain; GH19, glycohydrolase family 19; SLT, soluble lytic transglycosylase; Ca 2+ , Ca 2+ -binding domain; AHH, putative nuclease domain. ( b ) Gene names of putative lipoprotein signal peptide-containing Xac immunity proteins (X-Tfis) and sequences of the putative lipoprotein signal peptides. All seven of these genes are upstream of, and potentially co-transcribed with, the neighbouring X-Tfe gene. Lipoprotein signal peptides are characterized by an N-terminal basic region (basic residues coloured blue), a central hydrophobic region (underlined) followed by an [LVI]-[ASTVI]-[AGS]-C lipobox motif (red) [68] . Also indicated are the positions of the putative translation initiation codons relative to those found in the original annotation of the Xac genome [69] . Full size image XAC2609 lyses PG and XAC2610 is its inhibitor To test the above hypothesis, we performed a set of in vitro experiments to determine whether XAC2609 has the predicted lysozyme-like activity. Purified recombinant XAC2609 is able to degrade PG from the Gram-positive Micrococcus luteus ( Fig. 2a ), reduces the optical density and introduces a marked lag in the growth curve of Bacillus subtilis cultures ( Fig. 2b ), and results in B. subtilis cell lysis ( Fig. 2d ). These activities are maintained in an XAC2609 fragment lacking the XVIPCD (XAC2609 (1–308) ; Fig. 2a ) but are not observed when using a mutant XAC2609 (1–308) in which glutamic acid 48 within the predicted active site of the GH19 domain was changed to alanine ( Fig. 2a,e ). We observed similar lytic activity against PG ( Fig. 2a ) and B. subtilis ( Fig. 2g ) for a second XVIP, XAC0466, that has a domain architecture similar to XAC2609 plus a PG amidase domain ( Fig. 1a ). Furthermore, the XAC2609 lytic activity is inhibited by the addition of XAC2610 ( Fig. 2a,b and f ). XAC2610 is a specific inhibitor of XAC2609 since it was not able to inhibit the lytic activities of XAC0466 or hen egg white lysozyme ( Fig. 2a ). We also observed that XAC2609 and XAC2610 can be co-immunoprecipitated from Xac cells ( Supplementary Fig. 1a ) and that XAC2610 interacts with the catalytic XAC2609 N-terminal domain but not with the XVIPCD domain in vitro ( Supplementary Fig. 1b ). Due to these characteristics, we will therefore now refer to XAC2609 as X-Tfe XAC2609 (for Xanthomonadaceae-T4SS effector) and to XAC2610 as X-Tfi XAC2610 (for Xanthomonadaceae-T4SS immunity protein). 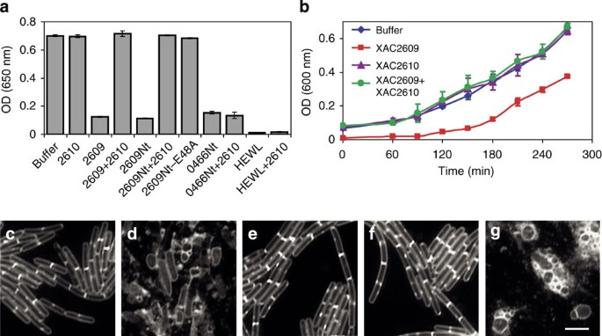Figure 2: X-TfeXAC2609is a peptidoglycan hydrolase and X-TfiXAC2610is its specific inhibitor. (a) Analysis ofM. luteuspeptidoglycan degradation, as determined by decreases in optical density (OD) at 650 nm of cell wall suspensions treated with purified proteins X-TfiXAC261055–267, 2610; full-length X-TfeXAC2609, 2609; X-TfeXAC2609(1–308)N-terminal fragment (residues 1–308), 2609Nt; X-TfeXAC2609(1–308_E48A)N-terminal fragment E48A mutant, 2609Nt-E48A; X-TfeXAC0466(1–475)N-terminal fragment (residues 1–475), 0466Nt; hen egg white lysozyme, HEWL. A suspension without the addition of any protein (buffer) is shown as a control. Error bars, s.d.;n=3. (b) Growth curves at 30 °C ofB. subtiliscells after incubation for 10 min without proteins (blue), with X-TfeXAC2609(red), X-TfiXAC2610(purple) or a mixture of both proteins (green; error bars, s.d.;n=3). (c–g) Fluorescence microscopy of membrane-labelledB. subtiliscells after incubation for 5 min withc, buffer;d, X-TfeXAC2609;e, X-TfeXAC2609(1–308_E48A);f, a X-TfeXAC2609-X-TfiXAC2610mixture;g, X-TfeXAC0466(1–475). Scale bar, 5 μm. Figure 2: X-Tfe XAC2609 is a peptidoglycan hydrolase and X-Tfi XAC2610 is its specific inhibitor. ( a ) Analysis of M. luteus peptidoglycan degradation, as determined by decreases in optical density (OD) at 650 nm of cell wall suspensions treated with purified proteins X-Tfi XAC2610 55–267 , 2610; full-length X-Tfe XAC2609 , 2609; X-Tfe XAC2609 (1–308) N-terminal fragment (residues 1–308), 2609Nt; X-Tfe XAC2609 (1–308_E48A) N-terminal fragment E48A mutant, 2609Nt-E48A; X-Tfe XAC0466 (1–475) N-terminal fragment (residues 1–475), 0466Nt; hen egg white lysozyme, HEWL. A suspension without the addition of any protein (buffer) is shown as a control. Error bars, s.d. ; n =3. ( b ) Growth curves at 30 °C of B. subtilis cells after incubation for 10 min without proteins (blue), with X-Tfe XAC2609 (red), X-Tfi XAC2610 (purple) or a mixture of both proteins (green; error bars, s.d. ; n =3). ( c – g ) Fluorescence microscopy of membrane-labelled B. subtilis cells after incubation for 5 min with c , buffer; d , X-Tfe XAC2609 ; e , X-Tfe XAC2609 (1–308_E48A) ; f , a X-Tfe XAC2609 -X-Tfi XAC2610 mixture; g , X-Tfe XAC0466 (1–475) . Scale bar, 5 μm. Full size image X-Tfi XAC2610 structure is similar to PG hydrolase inhibitors The X-Tfi XAC2610 protein does not share sequence similarity with any proteins of known function. We therefore determined the crystal structure of X-Tfi XAC2610 (55–267) (a fragment lacking the signal peptide, lipobox lipidation signal and a predicted unstructured region). Details of X-Tfi XAC2610 (55–267) crystallization, data collection and refinement are found in the Methods section and Supplementary Table 1 . X-Tfi XAC2610 has an N-terminal modified β-sandwich fold that includes a conserved integrin-like Ca 2+ -binding loop and an intramolecular disulfide bond, connected via a single α-helix to a C-terminal domain made up of an uncommon single-layer six-stranded antiparallel β-sheet ( Fig. 3a ). A more detailed description of the X-Tfi XAC2610 structure, including the Ca 2+ -binding loop and its semblance to a β-propeller fragment, is presented in Supplementary Fig. 2 . 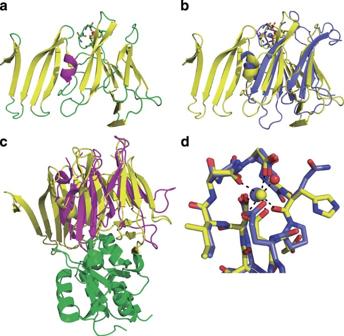Figure 3: X-TfiXAC2610is structurally similar to peptidoglycan hydrolase inhibitors. (a) Ribbon representation of the X-TfiXAC2610model (residues 55–267). A Ca2+ion and Ca2+-coordinating residues are shown as a sphere and sticks, respectively. (b) Superposition of X-TfiXAC2610(yellow) and PliI (light blue, PDB code 3OD9, ref.26). (c) Superposition of X-TfiXAC2610(yellow) and Tsi1 (pink). Tse1, the hydrolase inhibited by Tsi1, is shown in green in the Tsi1–Tse1 complex structure (PDB accession code 3VPJ, ref.27). Stereo versions ofbandccan be found inSupplementary Fig. 4. (d) Superposition of the X-TfiXAC2610and PliI ion-binding sites. Dashed lines show the pentagonal bipyramidal coordination of Ca2+in X-TfiXAC2610. The sticks colouring scheme forbanddare: C, yellow in X-TfiXAC2610and light blue in PliI; O, red; N, blue; Ca2+, yellow sphere; coordinating water, red sphere; Na+, light blue sphere. Search for structural similarities were performed using the Dali server60. The r.m.s.d., fraction of the chain for the superposition and % sequence identity of X-TfiXAC2610and Tsi1 are 3.4 Å, 82% and 7% respectively. For the superposition of X-TfiXAC2610and PliI, these values are 3.7 Å, 78% and 12% respectively. Supplementary Figure 3 presents small-angle X-ray scattering data that is consistent with a monomeric structure in solution. What is most interesting about the X-Tfi XAC2610 structure is that among its closest topological homologues are the periplasmic I-type lysozyme inhibitor PliI [25] , [26] ( Fig. 3b ) and the P. aeruginosa immunity protein Tsi1 ( Fig. 3c ) that inhibits the lytic PG DL-endopeptidase activity of its cognate T6SS effector protein Tse1 (refs 7 , 27 ; see also Supplementary Fig. 4 ). This topological similarity includes the superposition of the ion-binding sites of the X-Tfi XAC2610 and PliI proteins ( Fig. 3d ; Supplementary Fig. 4a ). The above in vitro and structural results show that X-Tfi XAC2610 is in fact the cognate immunity protein of the X-Tfe XAC2609 PG hydrolase toxin. Figure 3: X-Tfi XAC2610 is structurally similar to peptidoglycan hydrolase inhibitors. ( a ) Ribbon representation of the X-Tfi XAC2610 model (residues 55–267). A Ca 2+ ion and Ca 2+ -coordinating residues are shown as a sphere and sticks, respectively. ( b ) Superposition of X-Tfi XAC2610 (yellow) and PliI (light blue, PDB code 3OD9, ref. 26 ). ( c ) Superposition of X-Tfi XAC2610 (yellow) and Tsi1 (pink). Tse1, the hydrolase inhibited by Tsi1, is shown in green in the Tsi1–Tse1 complex structure (PDB accession code 3VPJ, ref. 27 ). Stereo versions of b and c can be found in Supplementary Fig. 4 . ( d ) Superposition of the X-Tfi XAC2610 and PliI ion-binding sites. Dashed lines show the pentagonal bipyramidal coordination of Ca 2+ in X-Tfi XAC2610 . The sticks colouring scheme for b and d are: C, yellow in X-Tfi XAC2610 and light blue in PliI; O, red; N, blue; Ca 2+ , yellow sphere; coordinating water, red sphere; Na + , light blue sphere. Search for structural similarities were performed using the Dali server [60] . The r.m.s.d., fraction of the chain for the superposition and % sequence identity of X-Tfi XAC2610 and Tsi1 are 3.4 Å, 82% and 7% respectively. For the superposition of X-Tfi XAC2610 and PliI, these values are 3.7 Å, 78% and 12% respectively. Full size image X-Tfe secretion is T4SS dependent and requires a XVIPCD We next tested whether X-Tfe XAC2609 is secreted in a manner dependent on the Xac T4SS. For this, we employed Xac Δ virD4 and Δ virB7 mutants, both of which are expected to abolish secretion of all T4SS substrates since VirD4 is the coupling protein required for recognition of T4SS substrates [2] and deletion of the Xac virB7 gene results in the disappearance of not just VirB7 but also VirB9 and VirB10 (ref 21 ), the principal components of the T4SS core complex [28] . Fig. 4a (top row) and Fig. 4b show that when Xac cells are spotted on nitrocellulose filters layered on Luria-Bertani (LB) agar plates, allowed to grow for 12 h and the cells washed away, we could not detect any secreted X-Tfe XAC2609 bound to the membrane since the background immunofluorescence signals of all Xac strains alone are the same as that observed for the Δ xac2609 mutant. However, extracellular X-Tfe XAC2609 is detected when wild-type (WT) Xac cells are mixed with an equal number of E. coli cells before spotting ( Fig. 4a , bottom row and Fig. 4b ). Moreover, E. coli -induced X-Tfe XAC2609 secretion is abolished in the Δ virD4 and Δ virB7 strains and restored when plasmids for expression of VirD4 or VirB7 proteins are introduced in these strains ( Fig. 4a,b ). These results show that X-Tfe XAC2609 is secreted by Xac on contact with E. coli cells in a T4SS-dependent manner. X-Tfe XAC2609 secretion is dependent on its XVIPCD since extracellular X-Tfe XAC2609 could only be detected in the experiments using a Xac Δ xac2609 mutant carrying a plasmid expressing full-length X-Tfe XAC2609 but not in mutant strains carrying empty plasmid or a plasmid that directs the expression of an X-Tfe XAC2609 fragment lacking the XVIPCD ( Fig. 4a,b ). Detection of extracellular X-Tfe XAC2609 in these experiments is not due to E. coli -induced Xac lysis since all Xac strains (except the uncomplemented Δ xac2609 mutant), including both Δ virD4 and Δ virB7 , produce intracellular X-Tfe XAC2609 ( Fig. 4c ). 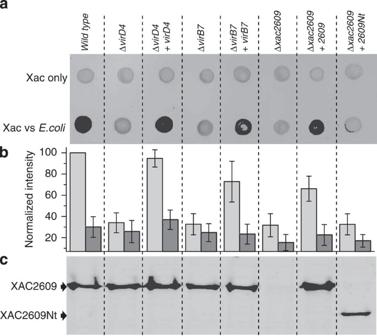Figure 4: X-TfeXAC2609secretion requires a XVIPCD, a functional T4SS and is stimulated by co-culture withE. colicells. (a) Xac cells only (top row) or 1:1 Xac:E. colimixtures (bottom row) were spotted on nitrocellulose filters layered on LB agar plates, allowed to grow for 12 h, the cells washed away and bound X-TfeXAC2609was immunodetected. The Xac wild-type (WT) strain (carrying pBBR-5GFP and empty pBRA vector) and the derived mutants (ΔvirD4, ΔvirB7and Δxac2609) and complemented strains (ΔvirD4+virD4, ΔvirB7+virB7, Δxac2609+xac2609and Δxac2609+xac2609Nt(X-TfeXAC2609N-terminal fragment)) used are indicated above each lane. (b) Integrated infrared fluorescence intensity of X-TfeXAC2609immunodetection from seven independent experiments similar to those represented inafor Xac only (dark bars) and Xac:E. colimixtures (light bars). Intensities were normalized to those measured for the WT Xac:E. colimixture. Error bars, s.d. (c) Western blot detection of total cellular X-TfeXAC2609produced by Xac strains used ina. The full blot is shown inSupplementary Fig. 9. Figure 4: X-Tfe XAC2609 secretion requires a XVIPCD, a functional T4SS and is stimulated by co-culture with E. coli cells. ( a ) Xac cells only (top row) or 1:1 Xac: E. coli mixtures (bottom row) were spotted on nitrocellulose filters layered on LB agar plates, allowed to grow for 12 h, the cells washed away and bound X-Tfe XAC2609 was immunodetected. The Xac wild-type (WT) strain (carrying pBBR-5GFP and empty pBRA vector) and the derived mutants (Δ virD4 , Δ virB7 and Δ xac2609 ) and complemented strains (Δ virD4 + virD4 , Δ virB7 + virB7 , Δ xac2609 + xac2609 and Δ xac2609 + xac2609Nt (X-Tfe XAC2609 N-terminal fragment)) used are indicated above each lane. ( b ) Integrated infrared fluorescence intensity of X-Tfe XAC2609 immunodetection from seven independent experiments similar to those represented in a for Xac only (dark bars) and Xac: E. coli mixtures (light bars). Intensities were normalized to those measured for the WT Xac: E. coli mixture. Error bars, s.d. ( c ) Western blot detection of total cellular X-Tfe XAC2609 produced by Xac strains used in a . The full blot is shown in Supplementary Fig. 9 . Full size image The Xac T4SS confers an advantage in growth competition experiments We then asked whether the T4SS confers a competitive advantage to Xac in growth competition experiments against other bacterial species. While there are no significant differences in the growth curves of the Xac WT and Δ virD4 and Δ virB7 mutant strains in liquid culture or on semi-solid media ( Supplementary Fig. 5 ), when Xac cells carrying a plasmid for the expression of cyan fluorescent protein (CFP) and E. coli cells expressing yellow fluorescent protein (YFP) were mixed and allowed to grow together as a co-culture on agar plates, we observed a significant increase in both the number and the size of the yellow E. coli colonies/zones in the cyan background of the Xac Δ virB7 strain when compared with that of the Xac WT strain ( Fig. 5a,b ). Xac competitiveness is recovered when the VirB7 protein is expressed in the Δ virB7 strain ( Fig. 5c ). The same phenomenon was observed in competition experiments using Xac Δ virD4 and Δ virB7 mutants expressing green fluorescent protein (GFP) and non-fluorescent E. coli ( Supplementary Fig. 6a ). Furthermore, after 38 h of co-culture growth, the Xac/ E. coli ratio is two orders of magnitude lower when Xac Δ virB7 strain is used, as compared with when the Xac WT strain or Xac ΔvirB7 strain carrying a plasmid for VirB7 expression are used ( Fig. 5d ). To further test whether T4SS mediates it effects in a contact-dependent manner, we placed a 0.2-μm pore filter between Xac and E. coli cells. Interestingly, the T4SS-dependent growth defect of Xac Δ virB7 and Δ virD4 mutant strains completely disappeared under this condition ( Supplementary Fig. 6b ), showing that direct contact is required for this T4SS function. Xac competitiveness against Chromobacterium violaceum , another Gram-negative species from a different bacterial class (Betaproteobacteria), was also observed to be T4SS dependent in the experiments similar to those shown in Fig. 5 ( Supplementary Fig. 7 ). 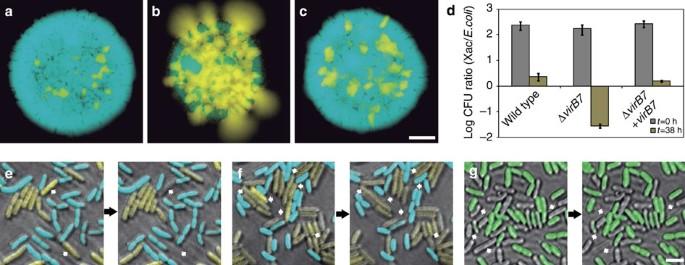Figure 5: Xac killsE. colicells in a T4SS-dependent manner. (a–c) Xac cells carrying a plasmid for the expression of CFP (cyan) andE. coliDH5α cells expressing YFP (yellow) were mixed at a 80:1 ratio, spotted on agar plates and allowed to grow together as a co-culture. The images show fluorescence emitted from the resultant colonies. Xac strains used were:awild-type (WT);bΔvirB7;cΔvirB7strain carrying a plasmid for VirB7 expression. Scale bar fora–c, 1 mm. (d) Ratio of the number of viable Xac andE. colicells in experiments similar to those shown ina–cafter 0 and 38 h of co-culture growth. Xac WT, ΔvirB7strain and theΔvirB7strain with ectopic VirB7 expression (ΔvirB7+virB7) were used. Error bars represent the s.d. of three experiments. (e–g) Superposition of brightfield and fluorescence microscopy images of single fields obtained after adding, to a thin agarose surface, mixtures containing equal amounts ofE. coliand (e) Xac WT, (f) ΔvirB7strain carrying a plasmid for VirB7 expression and (g) ΔvirD4strain carrying a plasmid for VirD4 expression. In these experiments, Xac cells carry a plasmid for the expression of CFP (cyan,e–f) or GFP (green,g), whileE. colicells carry a plasmid that expresses YFP (yellow,e–f) or are non-fluorescent (g). Arrows indicateE. colicells that underwent lysis during the 5-min intervals between images. Similar results were observed in dozens of experiments of this kind. In comparison, death of Xac cells was very rarely observed. Scale bar fore–g, 3 μm. Figure 5: Xac kills E. coli cells in a T4SS-dependent manner. ( a – c ) Xac cells carrying a plasmid for the expression of CFP (cyan) and E. coli DH5α cells expressing YFP (yellow) were mixed at a 80:1 ratio, spotted on agar plates and allowed to grow together as a co-culture. The images show fluorescence emitted from the resultant colonies. Xac strains used were: a wild-type (WT); b Δ virB7 ; c Δ virB7 strain carrying a plasmid for VirB7 expression. Scale bar for a – c , 1 mm. ( d ) Ratio of the number of viable Xac and E. coli cells in experiments similar to those shown in a – c after 0 and 38 h of co-culture growth. Xac WT, Δ virB7 strain and the ΔvirB7 strain with ectopic VirB7 expression (Δ virB7 + virB7 ) were used. Error bars represent the s.d. of three experiments. ( e – g ) Superposition of brightfield and fluorescence microscopy images of single fields obtained after adding, to a thin agarose surface, mixtures containing equal amounts of E. coli and ( e ) Xac WT, ( f ) Δ virB7 strain carrying a plasmid for VirB7 expression and ( g ) Δ virD4 strain carrying a plasmid for VirD4 expression. In these experiments, Xac cells carry a plasmid for the expression of CFP (cyan, e – f ) or GFP (green, g ), while E. coli cells carry a plasmid that expresses YFP (yellow, e – f ) or are non-fluorescent ( g ). Arrows indicate E. coli cells that underwent lysis during the 5-min intervals between images. Similar results were observed in dozens of experiments of this kind. In comparison, death of Xac cells was very rarely observed. Scale bar for e – g , 3 μm. Full size image The Xac T4SS mediates bacterial killing The competitive increment conferred by the Xac T4SS could be the result of secretion of factors that inhibit the growth of competing bacterial species or that promote direct killing of targeted adjacent cells. To distinguish between these two hypotheses, we used time-lapse microscopy to observe individual cells in Xac/ E. coli co-cultures. Figure 5e–g shows micrographs of single fields obtained shortly after mixing equal amounts of Xac and E. coli cells on a thin agarose surface. While we frequently observed the rapid lysis of E. coli cells that were in direct physical contact with Xac WT cells ( Fig. 5e ), we did not observe these events when the Δ virB7 and Δ virD4 strains were used ( Supplementary Fig. 8 ). Xac killing of E. coli was restored using mutant strains carrying plasmids for VirB7 or VirD4 expression ( Fig. 5f,g ). Supplementary Movie 1 presents a series of images separated by 300-ms intervals that show that E. coli cell lysis is extremely rapid, with cells often bursting in a seemingly explosive manner in <1 s to a few seconds. By comparison, Xac cell lysis was very rarely observed in these experiments. The rapid and violent cell death that we observe contrasts with that which has been reported for T6SS-mediated killing by Pseudomonas aeruginosa , in which target cells change their morphology (cell rounding, blebbing and plasmolysis) over a period of many minutes before lysis [29] , [30] . We have provided evidence that the Xac T4SS, and by extension its homologues in other Xanthomonadaceae species, target toxins (X-Tfes or XVIPs) to bacterial cells, thereby providing Xanthomonas an advantage to survive in an environment populated by a number of different bacterial species in a manner similar to that recently described for several T6SSs [29] , [30] , [31] , [32] , [33] . Using the presence of a XVIPCD as search criteria, we have identified 500 potential X-Tfes in the public databases, of which all but two are derived from members of the Xanthomonadaceae family ( Table 1 ). Most species that code for a Xanthomonadaceae-like T4SS code for several X-Tfe proteins and, in most cases analysed so far, one X-Tfe gene is found next to the gene of a T4SS component with the remaining X-Tfe genes found spread throughout the genome. Many of these proteins carry domains that may work to kill or inhibit growth of other organisms. Especially abundant are lipase domains [34] and domains involved in binding or modification of PG, found exclusively in bacterial cell walls [35] : for example, PG-binding domain 1 (ref. 36 ), transglycosylase SLT [37] , peptidase M23 (ref. 38 ), GH19 (refs 22 , 39 ) and NlpC/P60 (refs 38 , 40 ) domains ( Table 1 ). Other examples are the Zeta toxin domain that produces an inhibitor of bacterial PG biosynthesis [41] , the AHH domain likely involved in killing bacteria via its putative nuclease activity [42] and DUF2235 (ref. 43 ), a putative hydrolase recently found to be present in T6SS effectors [44] ( Table 1 ). Both Zeta toxin and AHH domains are found in toxin–antitoxin systems where they are inhibited by specific immunity proteins [41] , [42] . Table 1 Domains found in 500 proteins containing XVIPCDs. Full size table It is important to note that of the 500 X-Tfes (XVIPs) analysed in Table 1 , a large majority has no recognizable domain other than the C-terminal XVIPCD. Therefore, by studying the XVIP repertoire, we can reasonably expect the number of activities of this newly characterized T4SS and its effectors to expand. The proposed general bacterial killing function for a large number of Xanthomonadaceae-T4SS effectors may have interesting biotechnological applications that lead to new drug targets and ways of fighting other pathogenic bacteria that cause disease in humans and plants. Furthermore, we speculate that some X-Tfes could provide defence against eukaryotic microbes that prey on Xanthomonads. Finally, Ho et al . [45] recently showed that P. aeruginosa uses its T6SS to attack neighbouring cells carrying a mating pair formation T4SS encoded by a conjugative plasmid. The initial speculation was that this T4SS-induced T6SS counterattack potentially blocks acquisition of parasitic foreign DNA. However, since we have now demonstrated that some T4SSs pose a more immediate lethal threat to neighbouring bacteria, many bacterial species may have been under much stronger evolutionary pressure to have evolved an automatic T6SS counterattack response. This immediately suggests the hypothesis that, since very few T4SS have been characterized to date, T4SS-mediated bacterial killing may not be restricted to the Xanthomonadaceae family, and may in fact be a more widespread phenomenon. Bacterial strains, growth conditions and cloning Bacterial strains, oligonucleotides and plasmids used in this study are described in Supplementary Table 2 . All strains were grown on LB or 2 × TY (2 × yeast extract and tryptone) media. Concentrations of the antibiotics used: 100 μg ml −1 ampicilin, 20 μg ml −1 gentamicin, 100 μg ml −1 spectinomycin, 15 μg ml −1 tetracycline, 100 μg ml −1 chloramphenicol and 30 μg ml −1 kanamycin. For generation of the Xac Δ xac2609 strain, ~1 kb of the upstream and downstream regions of the xac2609 gene were amplified by PCR from Xanthomonas citri subsp. citri strain 306 genomic DNA and the two fragments were ligated to produce an in-frame deletion, leaving only the region coding for the first 15 and last 12 codons. This sequence was then cloned into the BamHI restriction site of the pNPTS138 suicide vector (M. R. Alley, unpublished; described in Supplementary Table 2 ), thereby generating the pNPTS138-2609 plasmid. For generation of the Xac Δ virD4 strain, a DNA fragment including the virD4 gene plus 0.55 kb upstream and downstream sequences were amplified by PCR and cloned into the NdeI/HindIII sites of the pUC19 vector. The resulting pUC19-virD4 vector was digested with the SacI restriction enzyme; as the virD4 gene has three of these sites, the digestion and subsequent re-ligation of the plasmid removed an internal fragment of 0.75 kb of virD4 , generating the pUC19-ΔvirD4. This strategy removed 251 codons of the central region of the gene, leaving the first 256 and the last 50 codons of virD4 . This plasmid was digested with Spe I/ Sal I and the resulting DNA containing the virD4 gene fragment plus 0.55 kb upstream and downstream sequences was cloned into the pNPTS138, thereby generating the pNPTS138-virD4 plasmid. In-frame deletions in the virD4 and xac2609 genes were obtained by a two-step allelic exchange procedure as previously described for the virB7 gene [21] using the pNPTS138-2609 and pNPTS138-virD4 vectors. For complementation of Xac mutant strains, genes virB7 XAC2622 , virD4 XAC2623 and xac2609 (coding the full-length protein (residues 1–431) or its N-terminal domain (residues 1–306)) were cloned in the pBAD24-derived vector pBRA (M. Marroquin, unpublished; described in Supplementary Table 2 ), which contains an arabinose-induced promoter that is constitutively active in Xac. Genes virB7 , virD4 , xac2609 and xac2609Nt were amplified by PCR from Xac306 genomic DNA and PCR products were cloned directly into the NcoI/SalI sites of pBRA. A recombinant XAC2610 (GenBank accession code AAM37459 ) fragment consisting of residues 22–267 fused to an N-terminal His-tag (X-Tfi XAC2610 (His-22–267) ) and full-length XAC2609 (residues 1–431; X-Tfe XAC2609 (1–431) ; GenBank accession code AAM37458 ) were expressed as described previously [20] . In brief, DNA coding for residues 55–267 of XAC2610 (X-Tfi XAC2610 (55–267) ) and N terminus (residues 1–308; X-Tfe XAC2609 (1–308) ) and C terminus (residues 311–431; X-Tfe XAC2609 (311–431) ) fragments of XAC2609 were amplified by PCR from Xac genomic DNA and cloned into the pET11a plasmid (Novagen) using the NdeI and BamHI cloning sites. The pET11a-XAC2609 1–308 vector was used as a DNA template for the generation of the pET11a-XAC2609-E48A plasmid that codes for X-Tfe XAC2609 (1–308_E48A) (the X-Tfe XAC2609 (1–308) protein with a Glu 48 to Ala mutation), using the QuikChange Site-Directed Mutagenesis Kit (Agilent Technologies). DNA coding for the N-terminal fragment of XAC0466 (residues 1–475; X-Tfe XAC0466 (His-1–475) ; GenBank accession code AAM35357 ) was cloned into the pET28a vector using the NdeI and BamHI sites, expressing a protein fused to an N-terminal His-tag. All plasmids were confirmed by DNA sequence analysis. Protein expression and purification E. coli BL21(DE3)RP strain (Novagen) was used for the expression of the recombinant proteins. Cells were grown in 2 × TY at 37 °C and recombinant proteins were induced at mid-log phase for 3–4 h by the addition of 0.5 mM isopropyl-β-D-thiogalactoside. Cells were then harvested and lysed by sonication employing a Vibra-Cell VCX-500 instrument (Sonics & Materials Inc.). The first chromatographic purification step was performed with a Q-sepharose anion exchange column (GE Healthcare) for all X-Tfe XAC2609 and X-Tfi XAC2610 constructions. The second chromatographic step was an affinity purification using a nickel chelate column for X-Tfi XAC2610 (His-22–267) , a size exclusion purification with a 26/600 Superdex 75 column for X-Tfi XAC2610 (55–267) , X-Tfe XAC2609 (1–308) and X-Tfe XAC2609 (311–431) or a 26/600 Superdex 200 column for X-Tfe XAC2609 (1–431) and X-Tfe XAC2609 (1–308_E48A) . X-Tfe XAC0466 (His-1–475) was purified using a nickel chelate column. PG hydrolase activity assay Micrococcus luteus cell wall suspensions (Sigma) with an optical density at 650 nm (OD 650 nm ) of 0.7 (0.8 mg ml −1 ) in 50 mM sodium acetate (pH 5.0) and 2 mM CaCl 2 were incubated in triplicate for 20 min at 30 °C with the following treatments: (i) without proteins (buffer), (ii) with X-Tfi XAC2610 (55–267) , (iii) X-Tfe XAC2609 (1–431) , (iv) X-Tfe XAC2609 (1–308) , (v) X-Tfe XAC2609 (1–308_E48A) , (vi) X-Tfe XAC0466 (His-1–475) , (vii) HEWL, (viii) X-Tfe XAC2609 (1–431) plus X-Tfi XAC2610 (55–267) , (ix) X-Tfe XAC2609 (1–308) plus X-Tfi XAC2610 (55–267) , (x) X-Tfe XAC0466 (His-1–475) plus X-Tfi XAC2610 (55–267) or (xi) HEWL plus X-Tfi XAC2610 (55–267) . X-Tfe XAC2609 -derived proteins, X-Tfe XAC0466 (His-1–475) and HEWL, were used at 1 μM concentration, while X-Tfi XAC2610 (55–267) was present at 2 μM. The reactions were stopped with the addition of 500 mM sodium carbonate. Cell wall degradation was monitored as a decrease in OD 650 nm . Bacterial growth inhibition assay Bacillus subtilis PY79 cells were grown in 2 × TY to log phase (OD 600 nm =0.5). Cells were harvested by centrifugation and resuspended to an OD 600 nm of 0.8 in 10 mM sodium acetate pH 5.0 and 1 mM MgCl 2 . Incubations were performed in triplicate for 10 min at 30 °C with only buffer or buffer containing 1 μM X-Tfe XAC2609 (1–431) or 2 μM X-Tfi XAC2610 (55–267) or 1 μM X-Tfe XAC2609 (1–431) plus 2 μM X-Tfi XAC2610 (55–267) . The bacteria were then diluted with nine volumes fresh 2 × TY medium and subsequent growth at 30 °C was monitored by measuring OD 600 nm . Bacillus subtilis lysis by X-Tfes Bacillus subtilis PY79 cells were grown in LB to OD 600 nm =0.5, harvested by centrifugation and resuspended to an OD 600 nm of 0.8 in 10 mM sodium acetate (pH 5.0), 1 mM MgCl 2 . Incubations were performed with only buffer or buffer containing (i) 1 μM X-Tfe XAC2609 (1–431) , (ii) 1 μM X-Tfe XAC2609 (1–308) , (iii) 1 μM X-Tfe XAC2609 (1–308_E48A) , (iv) 2 μM X-Tfi XAC2610 (55–267) , (v) 1 μM X-Tfe XAC2609 (1–431) plus 2 μM X-Tfi XAC2610 (55–267) , (vi) 1 μM X-Tfe XAC2609 (1–308) plus 2 μM X-Tfi XAC2610 (55–267) , (vii) 1 μM X-Tfe XAC0466 (His-1–475) or (viii) 1 μM HEWL. After 5 min of treatment at 23 °C, cells were centrifuged, washed, resuspended in 2 × TY and mounted on slides covered with a layer of 25% LB plus 1.5% agarose. Membranes were stained with FM1-43 or FM5-95 (Molecular Probes) at a final concentration of 1 μg ml −1 and the stained cells were analysed by fluorescence microscopy. Fluorescence microscopy Microscopy was carried out using a Nikon Eclipse Ti microscope equipped with filters for GFP (GFP-3035B-000-ZERO, Semrock), CFP (CFP-2432A-000-ZERO, Semrock), YFP (YFP-2427-000-ZERO, Semrock) and membrane visualization (Texas Red BrightLine set; TXRED4040-B, Semrock), a Plan APO VC Nikon 100 × objective (numerical aperture=1.4), a CFI Plan Apo Lambda Nikon 2 × objective and an Andor EMCCD i-Xon camera. The exposure times varied from 0.2 to 1 s. Images were processed and analysed using the programs Nis Elements (version 3.07; Nikon) and ImageJ ( http://rsbweb.nih.gov/ij/ ). Antibody production, immunoprecipitation and immunoblot Rabbit polyclonal antibodies were produced against X-Tfe XAC2609 (1–431) and X-Tfi XAC2610 (His-22–267) . Xac total cell lysates from WT and ΔvirB7 XAC2622 (ΔB7) strains were used for immunoprecipitation experiments with pre-immune serum or anti-X-Tfi XAC2610 serum (1:1,000 dilution), followed by immunoblots with anti-X-Tfe XAC2609 and anti-X-Tfi XAC2610 antibodies (1:1,000 dilution), performed as previously described [21] . Pre-immune serum, from the same animal later immunized with X-Tfi XAC2610 , was used as a negative control. Fluorescence spectroscopy Fluorescence assays were measured employing AVIV ATF-105 and Hitachi F-4500 fluorometers. Qualitative protein–protein interaction assays were carried out using 1 μM protein alone (X-Tfi XAC2610 (55–267) , X-Tfe XAC2609 (1–431) , X-Tfe XAC2609 (1–308) and X-Tfe XAC2609 (311–431) ) or combinations of X-Tfi XAC2610 (55–267) and one of the three X-Tfe XAC2609 fragments in 20 mM Tris-HCl pH 7.5, 50 mM NaCl, 3 mM EGTA and 4 mM CaCl 2 . Samples were pre-equilibrated at 25 °C for 2 min, excited at 295 nm (bandwidth of 2.5 nm) and fluorescence emission was recorded from 300 to 400 nm (bandwidth of 2.5 nm) at 0.2-nm intervals. The results of three experiments were averaged. Crystallization, data collection and processing Vapour diffusion sitting drop crystallization screens at 18 °C were performed for X-Tfi XAC2610 (His-22–267) , but no crystals were obtained. Two weeks incubation of this protein at room temperature produced an ~23 kDa proteolytic fragment that formed thin needle-like crystals. The N-terminal sequence of this fragment was determined by Edman degradation using a Sequenator model PPSQ-23 (Shimadzu) and MALDI-ToF measurements employing an Ettan MALDI-ToF mass spectrometer (GE Healthcare). The sequence was found to begin at residue 56 and mass spectroscopy analysis was consistent with a fragment consisting of X-Tfi XAC2610 residues 55–267. Recombinant X-Tfi XAC2610 (55–267) protein (400 μM dissolved in 10 mM Tris-HCl pH 7.0, 20 mM NaCl) was submitted to crystallization trials and crystals were observed after 2 weeks over a reservoir solution containing 100 mM Bis-Tris-HCl pH 5.5, 200 mM (NH 4 ) 2 SO 4 and 25% (w/v) PEG3350. Crystals were transferred to reservoir solution supplemented with 20% (v/v) glycerol and flash frozen at 100 K. X-ray diffraction data were collected using an in-house Rigaku MicroMax-007 HF microfocus rotating Cu anode generator (Institute of Chemistry, University of São Paulo) and the beamline W01B-MX2 of the Brazilian Synchrotron Light Laboratory (LNLS) [46] . The diffraction data were indexed, integrated and scaled using d*TREK [47] and HKL2000 (ref. 48 ). Data collection statistics are shown in Supplementary Table 1 . X-ray structure determination and refinement The crystal structure of X-Tfi XAC2610 (55–267) was determined by SIRAS (single isomorphous replacement with anomalous scattering) using crystals soaked for 5 min with reservoir solution supplemented with 20% (v/v) glycerol and a saturated solution of mercury acetate. The initial phase estimation was carried out using SHELXD [49] and autoSHARP [50] , followed by automatic model building by ARP/wARP [51] . The model was subsequently refined with the program Coot [52] with rounds of TLS [53] and restrained refinement in Refmac5 [54] from the CCP4 package [55] . Model quality was checked by Coot, Refmac5, MolProbity [56] , Rampage [57] and PROCHECK [58] . Clear electron density was visible for all residues except for the first four amino acids (residues 55–58) that were not, therefore, included in the model. The electron density of some specific exposed loops (residues 59–60, 139–143, 218–220 and 245–249) had a relatively lower signal-to-noise level but was sufficient to model their backbones with confidence. A total of 180 water molecules and a calcium ion were also modelled. The final model has R factor and R free of 0.200 and 0.241, respectively ( Supplementary Table 1 ). Figures were prepared using PYMOL ( http://www.pymol.org ) and protein topology schemes with TopDraw [59] . The coordinates of the X-Tfi XAC2610 (55–267) X-ray crystal structure were deposited in the PDB under accession code 4QTQ . Search for structural similarities were performed using the Dali server [60] . The Z -score, root mean squared deviation, number of residues superposed and fraction of the chain for the superposition of X-Tfi XAC2610 and Tsi1 are 6.5, 3.4 Å, 120 and 82%, respectively, and for the superposition of X-Tfi XAC2610 and PliI are 4.9, 3.7 Å, 95 and 78%. Small-angle X-ray scattering (SAXS) SAXS experiments were collected at the D11A-SAXS1 beamline at the LNLS in Brazil. The radiation wavelength was 1.55 Å and a Pilatus detector at 936 mm distance was used to give a scattering vector ( q =4 π / λ sin( θ ), where 2 θ is the scattering angle) ranging from 0.14 to 4.1 nm −1 . X-Tfi XAC2610 (55–267) at 3.34, 1.67 and 0.84 mg ml −1 dissolved in 20 mM Tris-HCl pH 7.5 and 100 mM NaCl was exposed in frames of 3 and 10 s, and only normalized data without significant radiation damage in the small q range were averaged to give the final scattering curve. Buffer scattering curves were collected and subtracted from the sample’s scattering curve, taking into account its attenuation. The scattering curves were normalized by the protein concentration to check for interference effects [61] or aggregation [62] over the SAXS curves. Guinier analysis was used to calculate the protein radius of gyration, R g, and to evaluate the monodispersity of the system. SAXS data analyses were performed using the ATSAS package [63] . The determination of the pair-distance distribution function, p ( r ), was conducted using the GNOM software [64] . After the p ( r ) calculation, 15 low resolution ab initio envelopes for X-Tfi XAC2610 (55–267) were generated with DAMMIN [65] and aligned and averaged using the program suite DAMAVER [66] . The normalized spatial discrepancy between the models was 0.562±0.011 and none were rejected. Comparisons of the scattering experimental data and X-ray protein models were performed using CRYSOL [67] . X-Tfe XAC2609 secretion analysis GFP-labelled Xac strains (Xac WT pBRA GFP, Xac ΔvirD4 pBRA GFP, Xac ΔvirD4 pBRA-virD4 GFP, Xac Δ virB7 pBRA GFP, Xac Δ virB7 pBRA-virB7 GFP, Xac Δ2609 pBRA GFP, Xac Δ2609 pBRA-2609FL GFP and Xac Δ2609 pBRA-2609Nt GFP; Supplementary Table 2 ) and E. coli BL21(DE3)RIL ArcticExpress were grown separately in 2 × TY to log phase (OD 600 nm of 1.0), centrifuged, washed and resuspended to OD 600 nm =2.0. Xac strains and E. coli were mixed at a 1:1 ratio. Xac alone or the mixtures (5 μl) were spotted onto a nitrocellulose transfer membrane (GE Healthcare). The filter was placed on LB agar media containing gentamicin and spectinomycin and maintained at 30 °C for 12 h. Cells were washed away with running water for 2 min, the filter was blocked in 10% non-fat milk and then incubated with anti-X-Tfe XAC2609 rabbit serum at 1:1,000 dilution. The primary antibody was detected using IRDye 800CW goat anti-rabbit IgG (LI-COR Biosciences) at 1:25,000 dilution. Membranes were scanned using an Odyssey CLx infrared imaging system (LI-COR Biosciences). Integrated fluorescence intensities with median background subtracted were quantified using the Image Studio Lite (version 4.0) software package, normalized to the values measured for the WT Xac: E. coli mixture, and the results from seven independent experiments averaged. Western blots of total cellular X-Tfe XAC2609 produced by the Xac strains were carried out with the same antibodies and documented using an Odyssey detection system as described above. Xanthomonas growth in liquid and solid media For analysis of Xac cell growth in liquid medium, the Xac WT, Δ virB7 and Δ virD4 strains were inoculated in triplicate in 2 × TY medium with a starting OD 600 nm of 0.05, grown for 2 days at 30 °C with agitation at 200 r.p.m. and the cell growth was monitored by measuring OD 600 nm and colony-forming unit (CFU) per ml at different time intervals. For analysis of cell growth on solid medium, 2.5 μl of Xac WT, Δ virB7 and Δ virD4 strains at OD 600 nm of 0.05 were plated onto LB agar medium. Colonies were resuspended in 1 ml of 2 × TY after 32, 53 and 74 h of growth and serial dilutions were plated on LB agar for CFU count. Interbacterial growth competition experiments Assays were performed in a manner similar to that described previously [7] , [33] . In brief, CFP-labelled Xac strains (Xac WT pUFR CFP, Xac Δ virB7 pUFR CFP and Xac Δ virB7 pUFR-virB7 CFP) and E. coli DH5α YFP ( Supplementary Table 2 ) were grown in 2 × TY to log phase (OD 600 nm =1.0), centrifuged, washed and resuspended to OD 600 nm =0.5. These Xac cells were then mixed with E. coli diluted at an 80:1 Xac: E. coli ratio. The mixtures were spotted on LB agar plates containing gentamicin and allowed to grow together as a co-culture at 30 °C. Fluorescence micrographs were collected after 48 h of incubation. Competition experiments of Xac cells (Xac WT GFP, Xac Δ virB7 GFP and Xac ΔvirD4 GFP; Supplementary Table 2 ) against C. violaceum were performed as above without antibiotic selection and analysed after 24 h of incubation. The results of competition experiments were quantified by determining the CFU of Xac and E. coli per colony of a co-culture initiated with a 180:1 Xac: E. coli mixture in which the initial Xac OD 600 nm =0.05. Xac strains used were Xac WT pUFR, Xac Δ virB7 pUFR and Xac Δ virB7 pUFR-virB7 and the E. coli strain was E. coli BL21(DE3)RIL ArcticExpress. Final Xac: E. coli ratios were calculated after 38 h of competition by resuspending the colony, performing serial dilution and plating the cells in LB agar media containing tetracycline for selection of E. coli and ampicillin for selection of Xac. Contact-dependent bacterial competition assays GFP-labelled Xac strains (Xac WT pBRA GFP, Xac ΔvirD4 pBRA GFP, Xac ΔvirD4 pBRA-virD4 GFP, Xac Δ virB7 pBRA GFP and Xac Δ virB7 pBRA-virB7 GFP; Supplementary Table 2 ) and E. coli BL21(DE3)RIL ArcticExpress were grown in 2 × TY to OD 600 nm =1.0, collected by centrifugation, washed and resuspended to OD 600 nm =2.0. Xac strains and E. coli were mixed at a 1:1 ratio. Xac alone or the mixtures were spotted onto a 0.22 μm polycarbonate membrane (Whatman) placed on LB agar plates containing gentamicin and spectinomycin and the gfp fluorescence emission from the Xac cells was documented after 24 h growth at 30 °C. In parallel, no-contact experiments were carried out by growing Xac cells on an intervening filter placed on top of an E. coli BL21(DE3)RIL ArcticExpress lawn grown on LB agar plates containing gentamicin and spectinomycin. The intervening filter prevents direct contact between Xac and E. coli cells. Microscopy analysis of Xac vs E. coli competition assays Xac strains (Xac WT pUFR CFP, Xac Δ virB7 pUFR CFP and Xac Δ virB7 pUFR-virB7 CFP or Xac WT pBRA GFP, Xac ΔvirD4 pBRA GFP and Xac ΔvirD4 pBRA-virD4 GFP; see Supplementary Table 2 ) and E. coli cells (DH5α YFP or BL21(DE3)RIL ArcticExpress) were grown in 2 × TY with appropriate antibiotics to OD 600 nm =1.0, centrifuged, washed, resuspended to OD 600 nm =2.0, mixed at a Xac: E. coli 1:1 ratio and 2 μl spotted onto an LB agarose pad (1.5% agarose in 25% LB medium). Interspecies competition was followed by fluorescence and brightfield microscopy. Brightfield time-lapse data were acquired every 0.3 s. Image analysis and movie edition were performed using ImageJ software, and Supplementary Movie 1 was processed at 20 frames per second (that is, each second of the movie is equivalent to 6 s of the experiment). Accession codes X-ray crystallographic coordinates and structure factors for X-Tfi XAC2610 have been deposited in the Protein Data Bank with accession code 4QTQ . How to cite this article: Souza, D. P. et al . Bacterial killing via a Type IV secretion system. Nat. Commun. 6:6453 doi: 10.1038/ncomms7453 (2015).